Optical hyperpolarization and NMR detection of129Xe on a microfluidic chip Optically hyperpolarized 129 Xe gas has become a powerful contrast agent in nuclear magnetic resonance (NMR) spectroscopy and imaging, with applications ranging from studies of the human lung to the targeted detection of biomolecules. Equally attractive is its potential use to enhance the sensitivity of microfluidic NMR experiments, in which small sample volumes yield poor sensitivity. Unfortunately, most 129 Xe polarization systems are large and non-portable. Here we present a microfabricated chip that optically polarizes 129 Xe gas. We have achieved 129 Xe polarizations >0.5% at flow rates of several microlitres per second, compatible with typical microfluidic applications. We employ in situ optical magnetometry to sensitively detect and characterize the 129 Xe polarization at magnetic fields of 1 μT. We construct the device using standard microfabrication techniques, which will facilitate its integration with existing microfluidic platforms. This device may enable the implementation of highly sensitive 129 Xe NMR in compact, low-cost, portable devices. Owing to the ease with which it may be placed in a non-equilibrium spin polarization state, 129 Xe gas has found extensive use in recent nuclear magnetic resonance (NMR) spectroscopy and magnetic resonance imaging (MRI) experiments, greatly enhancing the resultant NMR signal [1] . Furthermore, 129 Xe is extremely sensitive to its physiochemical environment, making it a valuable probe on length scales ranging from nanometres to metres [2] . It has enabled new applications ranging from the targeted detection of biomolecules [3] , [4] to perfusion imaging of the human lung [5] . However, the large-scale and non-portable nature of 129 Xe hyperpolarization hardware precludes its integration into microfluidic platforms, such as have found utility in the miniaturization of numerous analytical techniques [6] . Most 129 Xe optical polarizers have been designed to produce litre-sized volumes of polarized gas [7] , [8] . These systems, designed for clinical magnetic resonance imaging or the large-scale imaging of materials, are necessarily bulky, expensive and non-portable. Here, we present the fabrication and operation of a microfabricated source of hyperpolarized 129 Xe, suitable for the low-cost, power-efficient production of polarized gases and integration with microfluidic systems [6] , [9] , [10] . Our device uses an effective pumping volume of 25 μl and 8 mW of pumping light to achieve 129 Xe polarizations >0.5% at gas flow rates of 5 μl s −1 , in the absence of any superconducting magnet. This represents a signal enhancement of ~200 over the room temperature thermal equilibrium polarizations achievable at the highest commercially available magnetic field of 23.5 T. Our device requires only standard microfabrication techniques [11] , benefiting from some of the known strengths of this technology [12] , and employs concurrent high-sensitivity optical magnetometry [13] to detect the 129 Xe NMR signal. Our results are relevant in light of recent innovations in NMR [14] , which include sensitivity enhancement through the use of optically hyperpolarized 129 Xe gas [2] and optical magnetometry [15] , and the development of microfluidic NMR methods [16] . Our device combines all of these technologies in a single chip and may enable the implementation of fully integrated 129 Xe NMR instrumentation in low-cost, portable and sensitive lab-on-a-chip devices. Microfabricated source of hyperpolarized 129 Xe The chip, fabricated from silicon and glass, consists of four chambers 1 mm thick and several millimetres wide connected by micro-channels, as shown in Fig. 1a . A fraction of the 129 Xe atoms in the pump chamber (see Fig. 1a ) becomes polarized through spin exchange collisions with optically pumped 87 Rb atoms at a pumping rate proportional to the 87 Rb polarization, P Rb , and the spin-exchange rate, R se = n Rb γ se ,with n Rb being the alkali atomic number density and γ se the 87 Rb- 129 Xe spin-exchange rate coefficient [17] . Under gas flow, polarized 129 Xe atoms exit the pump chamber and move through the connecting channel into the probe chamber. Except where stated otherwise, both larger 87 Rb atomic density and stronger laser illumination in the pump chamber ensure that the pumping rate of 129 Xe in the pump chamber is much larger than that in the probe chamber. 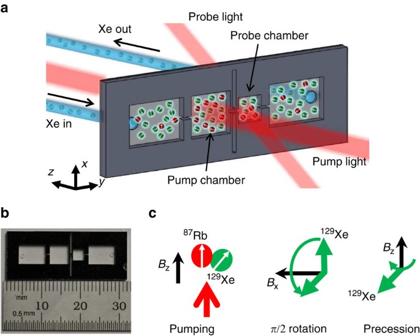Figure 1:The microfluidic chip129Xe polarizer. (a) A gas mixture containing 400 Torr N2and 200 Torr Xe in natural isotopic abundance (26.4%129Xe content) flows from a bulk gas manifold into the inlet chamber, through the pump and probe chambers, and out of the outlet chamber. The chip is loaded with 2 mg of87Rb metal (see Methods). Unpolarized129Xe atoms entering the pump chamber become polarized through spin exchange with optically pumped87Rb. The129Xe then moves downstream, passes through a microchannel into the probe chamber and eventually exits the device through the output chamber. Optical characterization of the129Xe polarization in the pump and probe chambers is carried out using the ensemble of87Rb atoms in each chamber asin situmagnetometers. (b) The silicon chip footprint is 3 cm × 1 cm, with a thickness of 1 mm. The dimensions of the pump and probe chambers are 5 mm × 5 mm × 1 mm and 3 mm × 3 mm × 1 mm, respectively, whereas the channel connecting the pump and probe chambers is 1 mm × 0.3 mm × 0.3 mm. Two tall, narrow grooves are etched from the middle of the chip to provide thermal isolation between the two sides of the device. (c) Pumping and probing sequence for129Xe. Pumping is carried out continually in the pump chamber in the presence of a longitudinal field ofBz=0.8 μT. Every 10–20 s, a transverse DC field of magnitude 5.3 μT is switched on for 4 ms to tip the129Xe atoms onto thex-yplane and initiate the129Xe precession about the longitudinal axis. Figure 1: The microfluidic chip 129 Xe polarizer. ( a ) A gas mixture containing 400 Torr N 2 and 200 Torr Xe in natural isotopic abundance (26.4% 129 Xe content) flows from a bulk gas manifold into the inlet chamber, through the pump and probe chambers, and out of the outlet chamber. The chip is loaded with 2 mg of 87 Rb metal (see Methods). Unpolarized 129 Xe atoms entering the pump chamber become polarized through spin exchange with optically pumped 87 Rb. The 129 Xe then moves downstream, passes through a microchannel into the probe chamber and eventually exits the device through the output chamber. Optical characterization of the 129 Xe polarization in the pump and probe chambers is carried out using the ensemble of 87 Rb atoms in each chamber as in situ magnetometers. ( b ) The silicon chip footprint is 3 cm × 1 cm, with a thickness of 1 mm. The dimensions of the pump and probe chambers are 5 mm × 5 mm × 1 mm and 3 mm × 3 mm × 1 mm, respectively, whereas the channel connecting the pump and probe chambers is 1 mm × 0.3 mm × 0.3 mm. Two tall, narrow grooves are etched from the middle of the chip to provide thermal isolation between the two sides of the device. ( c ) Pumping and probing sequence for 129 Xe. Pumping is carried out continually in the pump chamber in the presence of a longitudinal field of B z =0.8 μT. Every 10–20 s, a transverse DC field of magnitude 5.3 μT is switched on for 4 ms to tip the 129 Xe atoms onto the x - y plane and initiate the 129 Xe precession about the longitudinal axis. Full size image Optical detection of polarized 129 Xe Using the ensemble of 87 Rb atoms in the pump and probe chambers as magnetometers [13] , [18] , [19] sensitive to magnetic fields along the y -axis as defined in Fig. 1a , we detected the 129 Xe magnetization, and thus its polarization [20] , in each chamber as a function of the experimental conditions. The magnitude of the field B Rb sensed by 87 Rb due to 129 Xe magnetization M Xe is approximately [20] where μ 0 is the vacuum permeability, M Xe = μ Xe P Xe n Xe with μ Xe , P Xe and n Xe being the 129 Xe nuclear magnetic moment, polarization and atomic density, respectively. Here, κ 0 represents the enhancement factor due to the Fermi-contact interaction between the valence electron of 87 Rb and the 129 Xe nuclear spin [13] , [18] , [19] , [20] , [21] , previously measured to be κ 0 ≈500 (ref. 22 ). Measurement of the 129 Xe free-induction decay (FID) in each chamber is made with the magnetometers after rotating the 129 Xe longitudinal polarization along the z -axis into the transverse x - y plane with a transverse DC magnetic field pulse, as shown in Fig. 1c . 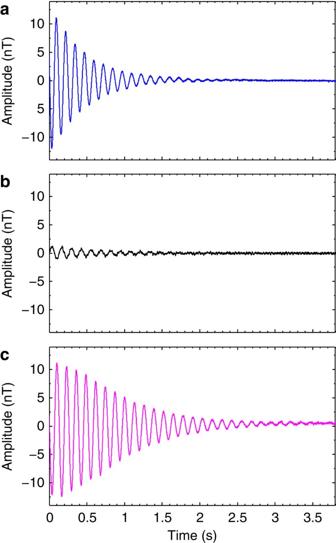Figure 2:Transport of polarized129Xe. (a) Free-induction decay (FID) of the transverse129Xe polarization in the pump chamber at a total gas flow rate of 3 μl s−1. (b) FID of polarized129Xe in the probe chamber with the pump light turned off. (c) FID of polarized129Xe in the probe chamber with the pump light turned on. Note that for this particular experiment the FID obtained inbis 180 degrees out of phase with that obtained in the pump chamber (a), due to the use of opposite-handed polarizing photons in the pump and probe chambers. Figure 2 demonstrates the efficient transport of polarized 129 Xe from the pump chamber to the probe chamber while the gas is flowing. Figure 2a shows the measured FID in the pump chamber, obtained by monitoring the transmitted power in the pump beam after the transverse field pulse. Figure 2b shows the measured FID in the probe chamber recorded with the pump beam blocked, so that there is no flow of polarized 129 Xe into the probe chamber. Under these conditions we observe a weak probe FID with amplitude of 1 nT, which we attribute to weak spin-exchange optical pumping (SEOP) of 129 Xe by the polarized 87 Rb in the probe chamber. Figure 2c shows that the probe FID changes significantly when the pump beam is unblocked; its amplitude increases and its phase changes by 180° to correspond to the amplitude and phase in the pump chamber observed in Fig. 2a . This indicates that the detected 129 Xe was polarized in the pump chamber and transported to the probe chamber by the flow of gas. Figure 2: Transport of polarized 129 Xe. ( a ) Free-induction decay (FID) of the transverse 129 Xe polarization in the pump chamber at a total gas flow rate of 3 μl s −1 . ( b ) FID of polarized 129 Xe in the probe chamber with the pump light turned off. ( c ) FID of polarized 129 Xe in the probe chamber with the pump light turned on. Note that for this particular experiment the FID obtained in b is 180 degrees out of phase with that obtained in the pump chamber ( a ), due to the use of opposite-handed polarizing photons in the pump and probe chambers. Full size image Characterization of 129 Xe polarization Next, we characterized the 129 Xe polarization in the pump and probe chambers as a function of total gas flow rate, alkali atomic density and pumping power. 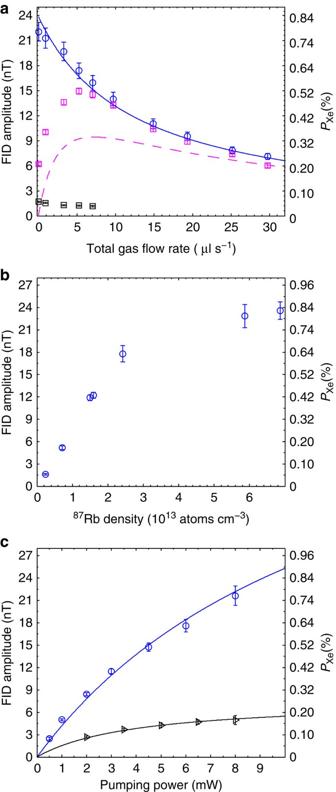Figure 3: Device characterization. (a)129Xe free-induction decay (FID) amplitude as a function of total gas flow rate in the pump chamber (blue circles), in the probe chamber with the pump light on (magenta squares), and with the pump light off (black squares). The solid line corresponds to a fit of the data using equation (2.1) withas a free parameter and withand(for details seeSupplementary Note 1). From the obtained value forand for a87Rb atomic density of 6 × 1013atoms cm−3in the pump chamber, which is estimated from the measured on-resonance optical depth (Methods), we estimate γse=1.7 × 10−16cm3s−1, in agreement with reported values for the spin-exchange rate coefficient due to87Rb-129Xe binary collisions17. The dashed line corresponds to the evaluation of equation (2.2) using the fitted value forand; this expression ignores87Rb-129Xe spin exchange and neglects the effects of diffusion, which can explain the discrepancy between the estimated line and the data at low flow rates. (b) Pump FID amplitude with no gas flow as a function of87Rb atomic density and (c) as a function of optical pumping power fornRb=6 × 1013atoms cm−3(blue circles) andnRb=1 × 1013atoms cm−3(black triangles). Incthe solid lines correspond to fits to the data using equation (1) and equation (2.1) withas a fitting parameter and using. The dependence of the Rb polarization was extracted from a fit to the measured shift in the129Xe Larmor frequency due to the87Rb magnetization as a function of pumping power (Supplementary Note 1). Error bars are given by 3σuncertainty in the fit for the FID amplitude. Figure 3a shows the amplitude of the FIDs and the corresponding 129 Xe polarization in the pump and probe chambers, which is estimated using κ 0 =500 (ref. 22 ) in equation (1), as a function of total gas flow rate. We observe that the polarization in the pump chamber decreases with flow, while in the probe chamber it builds up, peaks at a flow rate at which the influx of polarized 129 Xe is comparable with its spin-relaxation rate, and then follows the pump polarization. Figure 3: Device characterization. ( a ) 129 Xe free-induction decay (FID) amplitude as a function of total gas flow rate in the pump chamber (blue circles), in the probe chamber with the pump light on (magenta squares), and with the pump light off (black squares). The solid line corresponds to a fit of the data using equation (2.1) with as a free parameter and with and (for details see Supplementary Note 1 ). From the obtained value for and for a 87 Rb atomic density of 6 × 10 13 atoms cm −3 in the pump chamber, which is estimated from the measured on-resonance optical depth (Methods), we estimate γ se =1.7 × 10 −16 cm 3 s −1 , in agreement with reported values for the spin-exchange rate coefficient due to 87 Rb- 129 Xe binary collisions [17] . The dashed line corresponds to the evaluation of equation (2.2) using the fitted value for and ; this expression ignores 87 Rb- 129 Xe spin exchange and neglects the effects of diffusion, which can explain the discrepancy between the estimated line and the data at low flow rates. ( b ) Pump FID amplitude with no gas flow as a function of 87 Rb atomic density and ( c ) as a function of optical pumping power for n Rb =6 × 10 13 atoms cm −3 (blue circles) and n Rb =1 × 10 13 atoms cm −3 (black triangles). In c the solid lines correspond to fits to the data using equation (1) and equation (2.1) with as a fitting parameter and using . The dependence of the Rb polarization was extracted from a fit to the measured shift in the 129 Xe Larmor frequency due to the 87 Rb magnetization as a function of pumping power ( Supplementary Note 1 ). Error bars are given by 3 σ uncertainty in the fit for the FID amplitude. Full size image The dependence of the 129 Xe polarization in the pump chamber on the alkali atomic density, without gas flow, is shown in Fig. 3b . In our device, relaxation due to 129 Xe collisions with the glass walls is much faster than relaxation from spin-exchange collisions. Thus, equation (2.1) (see Methods) predicts a linear relationship between 129 Xe polarization and the 87 Rb- 129 Xe spin-exchange rate, which is proportional to the 87 Rb atomic density. This relationship, and a constant 87 Rb polarization, can explain the linear behavior of the 129 Xe polarization for low alkali atomic densities. At higher alkali densities the ensemble becomes optically thick and, given a finite amount of pumping power, the alkali polarization decreases. As a result the 129 Xe polarization no longer increases linearly with alkali density. This limitation can be observed in Fig. 3c , which shows the 129 Xe polarization in the pump chamber as a function of pumping power for low and high values of the optical depth OD 0 . At low optical thickness the 129 Xe polarization saturates, whereas for the larger optical depth it remains unsaturated at the highest applied optical powers. These results suggest that larger 129 Xe polarizations can be achieved by increasing both the 87 Rb density and pumping rate. The current polarizations achieved in our device are much lower than the near unity polarizations achieved in some large-scale polarizers [8] , [23] . However, as can be extrapolated from Fig. 3b and Fig. 3c , larger polarizations are in principle achievable in our device. We note that the 129 Xe relaxation of 1.6 s (see Supplementary Fig. 1 and Supplementary Note 1 ) observed in our system is 3 to 10 times faster than previously measured in sealed microfabricated cells with 1 mm 3 volume [24] , [25] . In this previous work, 129 Xe polarizations on the order of 5% were achieved using similar 87 Rb densities and slightly larger light intensities than those used in our device. These observations suggest room for improvement in future designs and motivate further study of the limitations of SEOP in microfabricated confinement volumes (see Supplementary Note 2 ). The combination of higher 87 Rb density, greater optical pumping power and improved relaxation times may allow for 129 Xe polarizations >5%. The current experiment is designed to produce a large magnetization signal at the expense of polarization through the use of a high 129 Xe partial pressure; the use of lower partial pressures is expected to trade off magnetization signal for increased polarization. An important figure of merit of a polarizer’s performance is its spin-transfer efficiency [1] ; for our device, the spin-transfer efficiency is ~0.0038, competitive with previous polarizers [23] , and only one order of magnitude smaller than the largest possible efficiency (see Supplementary Note 3 ). Another figure of merit is the ratio of the polarized atom flow rate to the optical pumping power. We obtain 0.45 μl s −1 W −1 for our device, again comparable to this quantity in large-scale polarizers [23] (see Supplementary Table 1 ). In this work, we employ the 87 Rb atoms as in situ detectors [13] , [18] , [19] of the 129 Xe magnetization and take advantage of the Fermi-contact interaction [13] , [18] , [19] , [20] , [21] to enhance the detection sensitivity to 129 Xe by a factor of ~500. This approach represents an important feature of our device that can be used to detect or monitor the 129 Xe polarization with high sensitivity at low magnetic fields in cases where the polarized gas can be cleanly extracted from the sample region. If the polarized gas cannot be extracted, as may occur if the gas has been dissolved in a liquid, for example, our device can be easily integrated with microfabricated magnetometers [26] placed outside of the pump and probe chambers. Microfabricated magnetometers have demonstrated sensitivities of 5 fT/√Hz over bandwidths of 100 Hz [26] , enough to detect the magnetic fields due to the currently produced 129 Xe polarization, and have been used to detect low-field NMR in microfluidics [27] . This approach may be useful for applications that are not compatible with the presence of alkali atoms in the microfluidic channels. We note that conventional glassblowing could also be used to make a compact system capable of producing small quantities of hyperpolarized gas. Compared with the microfabricated silicon-based system we describe here, we expect such a system to be somewhat larger and to require a higher pumping power, but likely to produce larger quantities of more highly polarized gas, due to the weaker wall relaxation and larger pumping volume. While the microfabricated chip described here is not particularly complicated to fabricate, requiring only simple lithography, etching and bonding, a compact glass-blown system may be simpler to implement in a laboratory setting to carry out scientific experiments on microfluidic systems. However, the microfabricated platform will likely be easier to integrate with other silicon-based microfluidic systems due to the common platform material. Microfabrication is likely to be most advantageous in an industrial setting where large numbers of devices might be manufactured. The possibility for large-scale parallel fabrication of devices would likely lead to lower production costs and higher reliability compared with conventional glass-blown systems. Our device, the first to hyperpolarize 129 Xe atoms in one chamber of a microfabricated device and optically interrogate them in another, will enable several new NMR applications without the need for immobile and expensive laboratory-scale instrumentation. We envision the development of portable high-density microfluidic arrays of xenon biosensors for the analysis of complex mixtures [4] , [16] , [28] in confined spaces such as micro-scale chemical reactors, or where access to hyperpolarized 129 Xe produced by large-scale polarizers is impractical, such as in field applications. In such applications, our device would produce hyperpolarized 129 Xe for dissolution into a liquid through use of a microfluidic gas-liquid mixer [29] . The NMR-encoded 129 Xe might be removed from the liquid through a microfluidic analogue of a superhydrophobic thin film [30] and then detected in situ with our integrated magnetometer, enabling extremely high chemical sensitivity, or detected ex situ with a physically separate chip-scale atomic magnetometer. Additional experiments suggested for large-scale 129 Xe polarizers [14] might also benefit from implementation on our portable, inexpensive device. Microfluidic chip fabrication The device consists of a 3 cm × 1 cm × 1 mm silicon chip. Deep reactive-ion etching (DRIE) is used to etch four holes of 1 mm depth to form the input, pump, probe and output chambers, as well as the channels connecting the input and output chambers to the pump and probe chambers, respectively. The channel connecting the pump and probe chamber is etched in a subsequent DRIE step. The device is sealed by anodically bonding two slides of borosilicate glass onto the top and bottom surfaces of the silicon chip. The lateral dimensions of the pump and probe chambers are 5 mm × 5 mm and 3 mm × 3 mm, respectively; they are connected by a 1 mm long × 300 μm wide × 300 μm deep channel. Before being bonded to the chip, one of the glass slides is drilled with holes situated in line with the input and output chambers, through which gas enters and exits the cell. Two 1/8″ VCR glands are glued onto the glass slide above the holes to allow connection of the cell to a gas manifold. The chip is filled with isotopically enriched 87 Rb vapour, produced by the chemical reaction of barium azide and 87 Rb chloride [31] within the input and output chambers as described in Supplementary Note 4 . Experimental setup The chip is placed inside a two-layer magnetic shield and attached to a gas manifold as shown in Supplementary Fig. 2 . Fine control of the gas flow rate through the chip is achieved by a leak valve placed downstream from the chip. Two independently controlled laser beams, tuned to the D1 optical transition of 87 Rb at 794.7 nm, irradiate the pump and probe chambers. A distributed feedback laser provides the pump laser beam, whereas light produced by a vertical-cavity surface-emitting laser is used as the probe laser beam. For most of the experiments, the optical power of the pump laser beam was 8 mW, while that in the probe was 100 μW. A set of Helmholtz coils is used to provide transverse magnetic fields in the x and y directions, and a solenoid is used to provide a longitudinal magnetic field in the z -direction. The pump and probe chambers are AC heated using two independent sets of surface mount resistors attached to the cell. The temperature at the input and output chamber is measured using two thermistors that are in close contact with the windows of those chambers. The device operates over a range of temperatures from 120 to 150 °C. The 87 Rb atomic density in each chamber is characterized by measuring the optical absorption of the laser beams as their wavelengths are scanned across the D1 optical line of 87 Rb. From the measured on-resonance optical depth OD 0 , we calculate the atomic density using OD 0 = σ 0 n Rb l with l =1 mm being the length of the beam path inside the pump chamber and σ 0 =2 r e cf /Δ υ being the on-resonance optical cross section where r e =2.8 × 10 −13 cm is the classical electron radius, c is the speed of light in vacuum, is the oscillator strength of the D1 resonance and Δυ=8 GHz is the full-width at half-maximum of the optical line obtained from the fitted optical absorption spectrum. Model for the 129 Xe polarization The measurements of the 129 Xe polarization in the pump and probe chambers can be interpreted in light of a model of the form where the superscripts Pu and Pr indicate the pump and probe chambers, respectively, R wall is the 129 Xe spin-destruction rate due to collisions with the chamber walls and R flow is the inverse of the 129 Xe transit time through the chamber. These equations are useful for understanding some characteristics of our device and guide future designs. We note, though, that they neglect diffusion, which limits the estimates of equation (2.2) at low flow rates. For example, Fig. 3a demonstrates that, when no gas is flowing, the polarization in the probe chamber is larger when the pump laser is on than when it is off. We have performed experiments, which are described in Supplementary Note 5 , indicating that this is due to the transport of polarized 129 Xe through diffusion (see Supplementary Figs 3–5 ). Diffusion is expected to be a uniquely important process for polarization transport in microfluidic systems such as those described here, for which the diffusion length is considerably larger than the characteristic size of the chip. Atomic magnetometer response and FID estimates The optically pumped 87 Rb magnetometers utilized here are very similar to those discussed in refs 18 and 19 . The magnetometers are implemented by introducing a radio-frequency field with 7 kHz modulation frequency and 1 μT amplitude along the y -axis. The signals of the magnetometers are extracted by lock-in detection of the transmitted laser intensity at the modulation frequency. The measured noise floors for the pump and probe magnetometers were and , respectively, with a bandwidth of 40 Hz that is limited by the response of the lock-in amplifiers. This corresponds to a single-shot detection limit of a polarized ensemble of ~5 × 10 11 129 Xe atoms in each chamber. On resonance, the magnetometers respond linearly to magnetic fields along the y axis that are smaller than the resonance line-width ( at zero-light levels dominated by collisions with Xe atoms, and twice or larger with optical pumping). For each change in the device parameters, the linear response of the magnetometers was obtained by extracting the on-resonance slope of the magnetic response acquired by scanning the magnetic field along the y axis. We then used this slope to calibrate the amplitude of the FIDs in magnetic field units. We fit the FID signal in the pump chamber to a single exponentially decaying sinusoid, from which we extracted the amplitude, decay time constant and Larmor precession frequency of 129 Xe. We obtained estimates for the FID amplitude in the probe chamber by measuring the amplitude of the first peak and valley in the probe FID signal. Because transverse polarization is transferred from pump to probe chambers as the FID signals are being taken, nonexponential decay of the probe FID can occur, preventing the simple analysis of the data with a single time constant. How to cite this article: Jiménez-Martínez, R. et al. Optical hyperpolarization and NMR detection of 129 Xe on a microfluidic chip. Nat. Commun. 5:3908 doi: 10.1038/ncomms4908 (2014).